Biomimetic approach to the catalytic enantioselective synthesis of tetracyclic isochroman 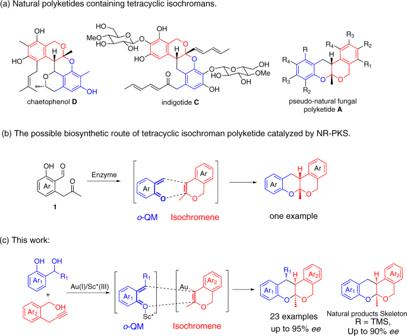Fig. 1: Background of tetracyclic isochromans and biomimetic design. aNatural polyketides containing tetracyclic isochromans.bThe possible biosynthetic route of tetracyclic isochroman polyketide catalyzed by NR-PKS.cThe bioinspired Au/Sc*catalyzed HDA reaction. Polyketide oligomers containing the structure of tetracyclic isochroman comprise a large class of natural products with diverse activity. However, a general and stereoselective method towards the rapid construction of this structure remains challenging due to the inherent instability and complex stereochemistry of polyketide. By mimicking the biosynthetic pathway of this structurally diverse set of natural products, we herein develop an asymmetric hetero-Diels–Alder reaction of in-situ generated isochromene and ortho -quinonemethide. A broad range of tetracyclic isochroman frameworks are prepared in good yields and excellent stereoinduction (up to 95% ee ) from readily available α -propargyl benzyl alcohols and 2-(hydroxylmethyl) phenols under mild conditions. This direct enantioselective cascade reaction is achieved by a Au(I)/chiral Sc(III) bimetallic catalytic system. Experimental studies indicate that the key hetero-Diels-Alder reaction involves a stepwise pathway, and the steric hindrance between in-situ generated isochromene and t -Bu group of Sc(III)/ N,N ’-dioxide complex is responsible for the enantioselectivity in the hetero-Diels–Alder reaction step. Tetracyclic isochromans, a type of polyketide oligomers [1] , [2] , [3] , are ubiquitously present in numerous natural products and bioactive molecules. For instance, Chaetophenol D was induced from chemically mediated epigenetic manipulation of fungal gene expression, exhibiting excellent anti -adenovirus activity [4] . Indigotide C and its isomer were biosynthesized by cultivation of Cordyceps indigotica , an entomopathogenic fungus, in the presence of suberoyl bis-hydroxamic acid, exhibiting good antibacterial activity [5] (see Fig. 1a ). Thus, the development of a general and stereoselective method towards a rapid construction is highly desirable. However, to our knowledge, such an effient methodology has not yet been established so far [6] , probably due to the inherent instability of tetracyclic isochroman polyketide and the difficulties in controlling the complex stereochemistry. Fig. 1: Background of tetracyclic isochromans and biomimetic design. a Natural polyketides containing tetracyclic isochromans. b The possible biosynthetic route of tetracyclic isochroman polyketide catalyzed by NR-PKS. c The bioinspired Au/Sc*catalyzed HDA reaction. Full size image As an important intermidiate, ortho -quinone methide ( o -QM) has caught much attention in the field of asymmetric catalysis [7] , [8] , [9] , [10] , [11] , [12] , [13] , [14] , [15] , [16] , [17] , [18] , [19] , [20] , [21] , [22] , [23] , [24] , [25] , [26] . Moreover, this highly reactive specie was proposed to be the diene intermidiate in the biosynthesis of several polyketide natural products via hetero-Diels–Alder (HDA) reaction. Asai and Oshima speculated a biosynthetic route of Indigotide C involving isochromene and o -QM intermidiates [5] . The same group developed a biosynthetic approach for the construction of a pseudo-natural fungal polyketide A by using 1 as substrate in 2015 [27] (see Fig. 1b ). The key of this method also lies in a HDA reaction of isochromene and o -QM which were heterologously biosynthesized by introducing the NR-PKS-encoding gene into Aspergillus oryzae . Inspired by this possible biosynthetic route of poliketide oligomer, we decided to exploit an artificial asymmetric catalytic system from the similar intermediates to build this complex structure. To the best of our knowledge, it is worth noting that there has been no report of biomimetic asymmetric catalytic HDA reaction involving o -QMs intermediates. The development of biomimetic HDA route for the synthesis of core structure of these natural products is of great significance to not only understand biosynthetic HDA reactions involving o -QM intermediates, but also expand the limitation of substrates catalyzed by Diels–Alderase enzymes [28] , [29] , [30] , [31] , [32] , [33] , [34] . The establishment of the enantioselective biomimetic polyketide oligomer synthesis requires the methods for the generation of isochromene and o -QM intermidiates and a catalyst capable of promoting the stereoselective HDA reaction. It is known that Au(I) complexes have been used in the cascade reactions [35] , [36] , [37] , [38] , [39] and could promote the intramolecular cyclization of benzyl alcohol-functionalized alkynes to isochromene intermediate [40] , [41] , and the o -QM intermidiate could be generated from the proper precursor in the presence of either acid or base. Recently, Au/Lewis acid bimetallic catalysis has been exploited to be a strategy to construct aminals and ketals via 5-exo-dig cyclization of alkynyl amides or alcohols and relay cycloaddition reactions with electrophiles [42] , [43] , [44] , [45] , [46] , [47] , [48] , [49] . Moreover, Feng’s group developed the first highly efficient asymmetric bimetallic Au(I)/chiral Ni(II) catalytic cascade reaction of α, β -unsaturated γ -keto esters with alkynyl amides and alcohols for the synthesis of spiroketals and spiroaminals in 2016 [50] . Kang and coworkers realized the same reaction by employing a Au(I)/chiral Rh(III) catalytic system two years later [51] . Inspired by these elegant works, we envisioned that a combination of a Au(I) catalyst and a chiral lewis acid catalyst might enable the HDA reaction of in-situ generated isochromene and o -QM to deliver the optically active tetracyclic isochromans, despite of that the acceptors of reported asymmetric Au/Lewis acid bimetallic catalysis were limited to α, β -unsaturated γ -keto esters, and the most of known asymmetric cascade reactions of alkynyl alcohols delivered spiro products rather than fused products [50] , [52] , [53] , [54] , [55] , [56] , [57] , [58] , [59] , [60] , [61] . 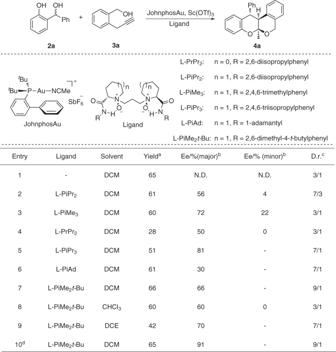Fig. 2: Optimization of the reaction. All reactions were carried out on a 0.1 mmol scale with 1 eq precursor ofo-QMs2a, 1.2 eq3a, 10 mol% of Sc(OTf)3, 11 mol% of ligand and 5 mol% of JohnphosAu in DCM (1 mL) at room temperature.aIsolated yield.bDetermined by chiral HPLC.cDetermined by by crude1H-NMR.dReaction temperature: 6 °C. In this work, we found a highly efficient Au(I)/chiral Sc(III) bimetallic catalytic system which could achieve asymmetric HDA reaction of in-situ generated isochromene and ortho- quinonemethide ( o -QM), and provided a diversity of tetracyclic isochromans in moderate to high yields and with high levels of diastereoselectivities and enantioselectivities (up to 95% ee ) (see Fig. 1c ). Studies commenced by screening effective precursors of o -QMs and the corresponding catalysts. We selected α -propargyl benzyl alcohol 3a as model substrate and JohnphosAu as the catalyst to generate isochromene intermidiate. 2-(Hydroxylmethyl) phenol 2a was chosen as the precursor of o -QM. Representative Lewis acids and Brønsted acids were investigated in the presence of 1.2 equivalent 3a and JohnphosAu catalyst (see the Supporting Information, Table S2 ). Sc(OTf) 3 was found to be the only efficient catalyst for this reaction, affording the HDA product 4a in 65% yield with 3/1 d.r. (Fig. 2 , entry 1). Subsequently, a series of other noble metal complexes such as Pd(II), Ag(I) and Au(I) complex were evaluated to generate isochromene intermidiate, but only (acetonitrile)Au-complex delivered the desire HDA products in good yield and no product was obtained by in-situ formed Au-complex (see the Supporting Information, table S2 ). Next, the screening of different types of chiral ligands for the purpose of achieving the asymmetric version of this reaction suggested that Feng ligands ( N,N’ -dioxide) showed unique activities in the asymmetric HDA reaction of in-situ generated isochromenes and o -QMs (Fig. 2 , entries 2-7). The use of ( S )-proline derived L-PrPr 2 resulted in lower diastereoselectivities and enantioselectivities than ( S )-piperidine derived L-PiPr 2 (Fig. 2 , entry 2 VS entry 4). More sterically hindered substituents at the para positions of aniline were beneficial to improve both diastereoselectivities and ee values (Fig. 2 , entries 5 and 7 VS entries 2 and 3) and aniline derived L-PiMe 2 t -Bu resulted in higher ee values than amantadine derived L-PiAd (Fig. 2 , entry 6 VS entry 7). The solvent screening suggested that the catalytic reactions were available in chlorinated solvents and DCM gave the best yield and selectivity (Fig. 2 , entries 7-9). Notably, after cooling to 6 °C, the ee value of the HDA product 4a was increased to 91% with little drop of yield (Fig. 2 , entry 10). Therefore, the optimized conditions involved the use of L-PiMe 2 t- Bu/Sc(OTf) 3 and JohnphosAu as catalysts in DCM at 6 °C (Fig. 2 , entry 10). Fig. 2: Optimization of the reaction. All reactions were carried out on a 0.1 mmol scale with 1 eq precursor of o -QMs 2a , 1.2 eq 3a , 10 mol% of Sc(OTf) 3 , 11 mol% of ligand and 5 mol% of JohnphosAu in DCM (1 mL) at room temperature. a Isolated yield. b Determined by chiral HPLC. c Determined by by crude 1 H-NMR. d Reaction temperature: 6 °C. Full size image Under optimized reaction conditions, the substrates scope of the reaction was examined. A series of aryl-substituted ortho- hydroxybenzyl alcohols 2a-i were tested with 3a as model α -propargyl benzyl alcohol (Fig. 3 ). Pleasingly, either electron-donating or electron-withdrawing substituents at the para- or meta- position of the benzene ring ( 2a-g ) were well tolerated, affording the corresponding poliketide oligomers in moderate yields and with good to excellent diastereoselectivities and enantioselectivities. In particular, the reactions of o -QMs with 2-naphthyl and 4-biphenyl substituents successfully afforded the desired products ( 4h , i ) in 76% and 60% yield with 90% and 84% ee respectively. However, ortho -substituted aryl groups have an extremely detrimental effect on the reactivity of this reaction probably due to the steric hinder effect. On the other hand, substituents at the quinone methide fragment were tolerated as well, and the corresponding adducts 4j-o were obtained in good to excellent enantioselectivities (81–89% ee ). Notably, alkyl-substituted o -QMs were also demonstrated to be acceptors amenable to the reaction protocol, giving rise to the corresponding products 4p-q with enantioselectivities up to 75% ee . 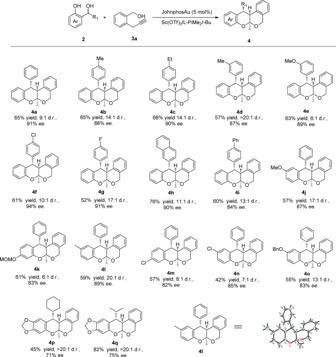Fig. 3: Substrates scope ofo-QMs. Unless otherwise noted, all reactions were carried out on a 0.2 mmol scale with 1.0 eq precursor of o-QMs2, 1.2 eq3a, 10 mol% of Sc(OTf)3, 11 mol% of L-PiMe2t-Bu and 5 mol% of JohnphosAu in DCM (2.0 mL) under 6 °C. Isolated yield for major diastereomer.eewas determined by chiral HPLC. D.r. was detected by crude1H-NMR. However, a variety of ortho -aminobenzyl alcohols could not afford the desired product probably due to the low reactivity of aza-o -quinone methide. The absolute configuration of 4 l was determined to be ( S,S,S ) on the basis of single crystal X-ray diffraction analysis. Fig. 3: Substrates scope of o -QMs. Unless otherwise noted, all reactions were carried out on a 0.2 mmol scale with 1.0 eq precursor of o-QMs 2 , 1.2 eq 3a , 10 mol% of Sc(OTf) 3 , 11 mol% of L-PiMe 2 t -Bu and 5 mol% of JohnphosAu in DCM (2.0 mL) under 6 °C. Isolated yield for major diastereomer. ee was determined by chiral HPLC. D.r. was detected by crude 1 H-NMR. Full size image Subsequently, we turned our attention to the substrates scope of α -propynyl benzyl alcohols by using o -QM precursor 2 h as substrate. As shown in Fig. 4 , a wide range of α -propynyl benzyl alcohols 3b-i bearing different substituted aryl groups reacted with 2 h quite well to form the corresponding poliketide oligomers 4r - 4y in good to moderate yields (43–72%) with excellent ee values (89–95%). In general, electron-donating groups furnished the poliketides 4r and 4 s in higher yields than those with electron-withdrawing substituents 4t-y , albeit in similarly high ee values. Cbz-protected α -propargyl benzyl amine 3j as well as various alkyl benzyl alcohol derivatives 3k-q was investigated in this cascade reaction under the optimized reaction conditions. 3j reacted with 2 h quite well to form the corresponding N- aza poliketide oligomer 5a in 63% yield, 1.5:1 d.r with 22% ee for major diastereoisomer and 15% ee for minor diastereoisomer. The reactions between 2 h and α -ethynyl benzyl alcohols 3k-l were carried out with L-PiAd as ligand and chiral spiro products 5b-c were isolated in 72–76% yield and 52–55% ee . 2-(Propynyl)phenol 3 m was also tolerated as well under the standard reaction condition and gave the corresponding chiral spiro product 5d in 31% yield with 37% ee . Moreover, alkyl benzyl alcohol 3o reacted with 2 h to form the product 5 f by 1,4-addition without annulation in 8 membered ring system likely due to the ring strain. It is worth mentioning that the reaction between 3n and 2 h was messy toward 7 membered ring system and poliketide oligomer 5e was isolated in 14% yield with 0% ee . Internal alkynes 3p-q were also demonstrated to be reactants amenable to the reaction protocol, giving rise to the corresponding products 5g-h in 39–41% yield with 53–55% ee . Hexynols 3s-t are unavailable substrates in this catalytic system. However, pentynol derivative 3r reacted quite well with 2 h to form the chiral spiro product 5i in 52% yield with 66% ee . Fig. 4: Substrates scope of α-propargyl benzyl alcohols. Unless otherwise noted, all reactions were carried out on a 0.2 mmol scale with 1 eq 2h , 1.2 eq 3 , 10 mol% of Sc(OTf) 3 , 11 mol% of L-PiMe 2 t -Bu and 5 mol% of JohnphosAu in DCM (2.0 mL) under 6 °C. Isolated yield for major diastereomer. ee was determined by chiral HPLC. D.r. was detected by crude 1 H-NMR. a 11 mol% of L-PiAd as ligand. Full size image To evaluate the synthetic potential of this protocol, the cascade reaction of 2 h and 3a was carried out on a gram scale under optimized reaction conditions with Au(I)/ N , N ′-dioxide-Sc(ΙΙΙ) complex. The corresponding product, tetracyclic isochroman poliketide oligomer 4 h , could be obtained with 52% yield, 9:1 d.r. and 90% ee (Fig. 5a ). In addition, derivatizations of product 4 were performed without loss of enantiopurity of the functionalized products. For example, the controllable selective cleavages of C-O bonds in poliketide 4d were carried out without any deterioration of enantiopurity (Fig. 5b ). In the presence of strong Lewis acid BF 3 •OEt, 4d was readily cleaved to the corresponding oxonium ion to furnish bioactive compound 6 which was reported to be an estrogen receptor degrader for treatment of ER+ breast cancers with good yield and complete diastereocontrol (Fig. 5b , black part). If TiCl 4 was used as strong Lewis acid instead of BF 3 •OEt, 4d was readily transformed to another oxonium ion and phenol 7 was obtained (Fig. 5b , blue part). Considering the structure of tetracyclic isochroman natural product, 8r (R = H) as a precursor of o -QM was tested in the asymmetric reaction with 2a , but no product was obtained. Unexpectedly, TMS substituted ortho -hydroxybenzyl alcohol 8 s gave the product 9a with the skeleton of natural product directly under standard conditions in 90% ee albeit with somewhat eroded yield (Fig. 5c ). Fig. 5: The gram scale experiment and transformations of product 4. a The gram scale experiment. b Reduction of product 4d . c Synthesis of analogue of pseudo-natural fungal polyketide A . Full size image As a key step toward establishing the basis for diastereo- and enantiocontrol in this cascade reaction of 1-(hydroxymethyl)-2-phenols 2 and α -propargyl benzyl alcohols 3 with the catalysis of Sc(ΙΙΙ)/Au(I), we endeavored to determine whether the HDA reaction of in-situ generated isochromene and ortho -quinonemethide proceeds via a concerted or stepwise pathway. To address this question, we investigated the carbon isotope effects for the [4 + 2] reaction between 2b and 3a using Singleton’s method at natural abundance [62] , [63] . When the reaction was stopped at 71% conversion, the 13 C ratio of each carbon in the recovered 3-methyl-1H-isochromene 10 to the same carbon in virgin 10 was measured using quantitative 13 C NMR. As shown in Fig. 6 , the only appreciable carbon isotope effect was observed at the 4-C-position of 10 , thus indicating that the HDA cycloaddition might proceed through a stepwise mechanism to form adducts. Fig. 6: Carbon isotope effects (R/R 0 ) calculated for 3a . The carbon valued in bold was taken as the internal standard. Full size image In order to investigate the role of the Au-complex in this enantioselective cascade reaction, we investigated the hetero-Diels-Alder reaction between o -QMs precursor 2b and 3-methyl-1H-isochromene 10 with or without the participation of Au-complex (Fig. 7 , entry 2 and 3). Two catalytic reactions afforded the tetracyclic isochroman poliketide oligomer 4b in similar yield, d.r. and ee values comparing to the cascade reaction between 2b and 3a (Fig. 7 , entry 1), which suggests that 10 may be the real active intermediate in the [4+2] cycloaddition and Au-complex may not participate in the control of the enantioselectivity. Fig. 7: Controlled experiments. 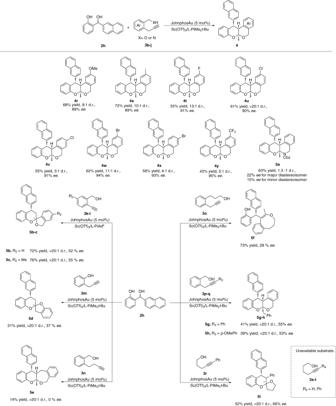Fig. 4: Substrates scope of α-propargyl benzyl alcohols. Unless otherwise noted, all reactions were carried out on a 0.2 mmol scale with 1 eq2h, 1.2 eq3, 10 mol% of Sc(OTf)3, 11 mol% of L-PiMe2t-Bu and 5 mol% of JohnphosAu in DCM (2.0 mL) under 6 °C. Isolated yield for major diastereomer.eewas determined by chiral HPLC. D.r. was detected by crude1H-NMR.a11 mol% of L-PiAd as ligand. Unless otherwise noted, all reactions were carried out on a 0.2 mmol scale with 1 eq 2b , 1.2 eq 3a or 10 , 10 mol% of Sc(OTf) 3 , 11 mol% of L-PiMe 2 t -Bu and 5 mol% of JohnphosAu in DCM (2.0 mL) under 6 °C. Full size image Based on the reported X-ray structure of the N,N ’-dioxide Sc III complex [64] and the absolute configuration of the product 4 as well as the results of control experiments, we proposed a catalytic model for the Au/Sc*catalyzed HDA reaction (Fig. 8 ). A complex with octahedral geometry as the transition state is formed by coordinating L-PiMe 2 t- Bu and o -QMs to Sc III center. The enol attack takes place from the less hindered Si face of the o- QMs to form the first chiral center in the benzylic position of o -QM skeleton (Fig. 8 , 1a VS 1b). Subsequent oxygen anion attack to oxonium ion affords the desired optical tetracyclic isochroman from Si face, while the Re face of the oxonium ion is shielded by the N,N ’-dioxide (Fig. 8 , 1c VS 1d). Fig. 8: Proposed stereochemical models. a Favor transition state of first step. b Disfavor transition state of first step. c Favor transition state of second step. d Disfavor transition state of second step. Full size image In summary, we designed and developed the first asymmetric HDA reaction of in-situ generated isochromene and o -QM based on insights from the biosynthetic pathway of polyketide oligomer natural products. This direct enantioselective cascade reaction was achieved through a Au(I)/Sc(III) bimetallic catalytic strategy, affording a series of chiral tetracyclic isochromans from readily available α -propargyl benzyl alcohols and 2-(hydroxylmethyl) phenols under mild conditions. Importantly, this work demonstrates the potential utility of biomimetic synthesis in the development of reaction and expanding the limitation of substrates comparing to biosynthesis expansion, which encourages us to explore biomimetic catalytic reactions in the future. General experimental procedure of asymmetric cascade reaction To a 10-mL test-tube were sequentially added JohnphosAu (0.010 mmol, 7.7 mg), Sc(OTf) 3 (0.020 mmol, 9.8 mg), L-PiMe 2 t -Bu (0.022 mmol, 14.4 mg) and CH 2 Cl 2 (2.0 mL). The mixture stirred for 15 min. 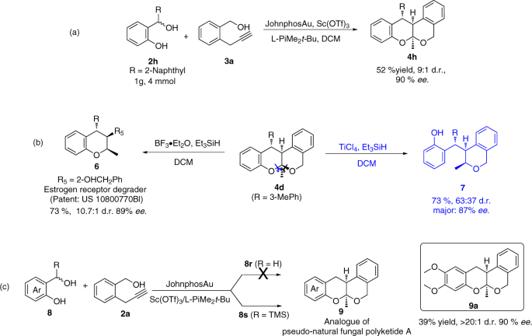Fig. 5: The gram scale experiment and transformations of product 4. aThe gram scale experiment.bReduction of product4d.cSynthesis of analogue of pseudo-natural fungal polyketideA. α -Propargyl benzyl alcohol 3 (0.3 mmol) and substrate 2 (0.2 mmol) were added in turn to the solution at 6 °C. The reaction mixture was monitored by TLC. Upon completion, the residual was purified by silica gel flash chromatography (petroleum ether:ethyl acetate, 20:1) to afford the desired product 4 . The racemic examples were prepared by the catalysis of Sc(OTf) 3 in r.t. Experimental procedure for synthesis of 6 Under Ar atmosphere, to a 10-mL test-tube were sequentially added 4d (0.4 mmol, 136.8 mg) (89% ee ), CH 2 Cl 2 (2.0 mL), Et 3 SiH (0.4 mmol, 46.4 mg) and BF 3 ·Et 2 O (0.2 mL) in 0 °C. Upon completion (2 h) the residual was purified by silica gel flash chromatography (petroleum ether:ethyl acetate, 5:1) to afford the desired product 6 . Experimental procedure for synthesis of 7 Under Ar atmosphere, to a 10-mL test-tube were sequentially added 4d (0.2 mmol, 68.4 mg) (89% ee ), CH 2 Cl 2 (2.0 mL), Et 3 SiH (0.2 mmol, 23.2 mg) and TiCl 4 (0.1 mL) in 0 °C. 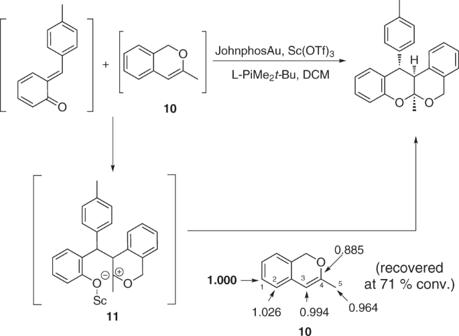Fig. 6: Carbon isotope effects (R/R0) calculated for3a. The carbon valued in bold was taken as the internal standard. 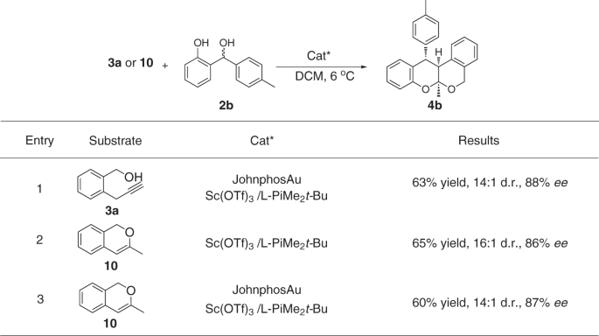Fig. 7: Controlled experiments. Unless otherwise noted, all reactions were carried out on a 0.2 mmol scale with 1 eq2b, 1.2 eq3aor10, 10 mol% of Sc(OTf)3, 11 mol% of L-PiMe2t-Bu and 5 mol% of JohnphosAu in DCM (2.0 mL) under 6 °C. 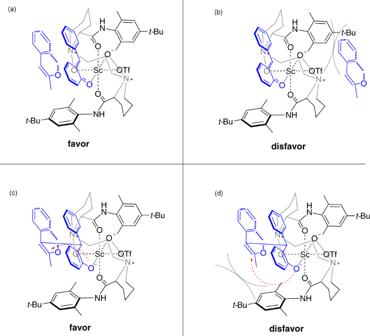Fig. 8: Proposed stereochemical models. aFavor transition state of first step.bDisfavor transition state of first step.cFavor transition state of second step.dDisfavor transition state of second step. Upon completion (2 h) the residual was purified by silica gel flash chromatography (petroleum ether:ethyl acetate, 5:1) to afford the desired product 7 .